Manipulating surface reactions in lithium–sulphur batteries using hybrid anode structures Lithium–sulphur batteries have high theoretical energy density and potentially low cost, but significant challenges such as severe capacity degradation prevent its widespread adoption. Here we report a new design of lithium–sulphur battery using electrically connected graphite and lithium metal as a hybrid anode to control undesirable surface reactions on lithium. Lithiated graphite placed in front of the lithium metal functions as an artificial, self-regulated solid electrolyte interface layer to actively control the electrochemical reactions and minimize the deleterious side reactions, leading to significant performance improvements. Lithium–sulphur cells incorporating this hybrid anodes deliver capacities of >800 mAh g −1 for 400 cycles at a high rate of 1,737 mA g −1 , with only 11% capacity fade and a Coulombic efficiency >99%. This simple hybrid concept may also provide scientific strategies for protecting metal anodes in other energy-storage devices. Although rechargeable lithium (Li) ion batteries (LIBs) are widely studied for application in portable electronic devices and vehicle electrification, they cannot store sufficient energy for the extended driving range required by electric vehicles [1] , [2] , [3] , [4] , [5] , [6] , [7] . Alternative energy-storage systems with much higher theoretical specific energy are needed [8] , [9] , [10] , [11] . Among these technologies, Li–sulphur (Li–S) batteries hold great promise [8] , [9] , [10] , [11] , [12] , [13] , [14] , [15] , [16] , [17] , [18] , [19] . Theoretically, a Li–S battery has a specific capacity and energy of 1,675 mAh g −1 and 2,600 Wh kg −1 , respectively, much higher than those of traditional LIBs. Sulphur is also of low cost, and is abundant and non-toxic, making this system attractive for large-scale applications. However, many obstacles in this system still need to be overcome for practical applications. The major issue associated with Li–S cells is the formation of soluble long-chain polysulphides during discharge/charge. The gradual loss of active mass from the cathode into the electrolyte and onto the Li metal anode leads to ‘shuttle reactions’, severe self-discharge, low efficiency and fast capacity decay on cycling, which are commonly observed in Li–S batteries. Various strategies have been employed to address the polysulphide shuttle challenges in Li–S cells. For cathodes, nanostructured hosts such as mesoporous carbon, graphene, carbon nanofibres [16] , [20] , [21] , [22] , [23] , [24] , [25] , [26] , oxygenated porous architectures [27] or conductive polymers have been used to trap sulphur [20] , [28] , [29] , [30] , [31] . One example is Nazar’s precise constraint of sulphur within a mesoporous carbon framework [16] . The use of an ordered mesoporous carbon composite provides both an electronic percolation path and an adequately controlled porosity that confines a significant portion of the electrochemically generated polysuphide species in the cathode. Other approaches focus on the electrolyte, including the selection of appropriate solvents [32] , [33] , dual electrolytes [34] , electrolyte additives [13] , [35] , [36] , [37] , [38] , [39] or solid-state electrolytes [40] . Scrosati and co-workers [17] , [41] , [42] used a gel-type polymer electrolyte membrane as a physical barrier to block the dissolved sulphide species within the cathode compartment and lessen the deleterious side reactions at the anode. Investigation of new binders [43] has also been reported in an attempt to improve the integrity of the electrode structure, facilitate electron transport and improve Li + ion diffusion [21] . In addition to the sulphur dissolution problem at the cathode, other studies suggest that continuous contamination of polysulphide species on the Li metal anode is equally, if not more severely, damaging to long-term cell performance, but this problem has received much less attention. For any rechargeable batteries employing Li metal as the anode, two major failure mechanisms are typically associated with the system. One is the uncontrolled dendrite formation [44] , whereas the other is the continuous evolution of a porous, or mossy, Li metal structure that lowers cell efficiency [45] . The former presents serious safety issues, particularly at high charging rates, whereas the latter continually erodes the anode. This chemical and electrochemical corrosion repeatedly exposes new Li surface area that further reacts with the electrolyte to form unstable solid-state electrolyte interface (SEI) layers, thus increasing internal cell resistance and accelerating capacity fade [22] , [23] , [24] , [25] . For Li–S batteries, where Li metal is coupled with sulphur cathode, the deposition/reduction of insoluble short-chain polysulphides on a Li anode partially mitigate the dendrite growth problem [33] , [46] . However, the problem of continuous Li erosion still exists and is compounded with the presence of dissolved polysulphides that also get involved in the continuous SEI formation [47] . Sion Power found that LiNO 3 , used as an electrolyte additive, helps minimize complicated deleterious reactions between polysulphides and Li, resulting in improved cell life [13] . Tarascon and colleagues [48] also reported that direct coating of the Li anode by sulphur effectively stabilizes the cycling of Li–S batteries. Other work also suggests that even a Li/Li 2 S 9 liquid cell can be cycled if an appropriate protective/passivation film can be formed on the Li metal anode [37] , [49] . A recent publication, monitoring the content of dissolved sulphur with cycling, further indicates that factors in addition to the dissolved sulphur may be the primary reason for the fast capacity fade in Li–S cells [50] . On the basis of the above considerations, further improvements in Li–S cell performance may be achieved by concentrating on advanced anode designs. We speculate that rather than simply using an electrolyte additive or a physical barrier (film) to protect the metal anode, it may be possible to design a completely different anode structure where the interfacial redox reaction is shifted away from the metal surface. To test this hypothesis, a compacted graphite film is connected with Li foil as an integrated anode and tested against a sulphur cathode [20] . 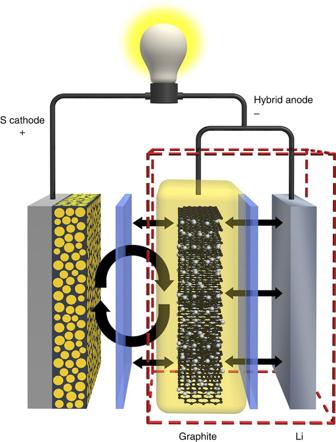Figure 1: Schematic of the hybrid anode design. Schematic of the hybrid anode design to manipulate the surface reactions on Li–S batteries. Figure 1 shows the schematic of proposed hybrid anode placed in a Li–S battery. The graphite/Li connected in parallel forms a shorted cell where the graphite is always lithiated at equilibrium and maintains a pseudo-equal potential with the Li metal. As such, it functions as an artificial SEI layer of Li metal that supplies Li + ions on demand, while minimizing direct contact between soluble polysulphides and the metal surface. Figure 1: Schematic of the hybrid anode design. Schematic of the hybrid anode design to manipulate the surface reactions on Li–S batteries. Full size image Cell configuration and cell performance In the hybrid anode design, a graphite film is placed between the Li foil and separator, and then electrically connected with the Li metal to form a parallel anode ( Fig. 1 ). Once immersed in the electrolyte, Li ions immediately intercalate into the graphite, which persists in the lithiated state because this hybrid anode is, in fact, a shorted cell. Using this anode concept, the hybrid Li–S cell delivers a reversible capacity of >900 mAh g −1 at 1,370 mA g −1 (~0.8 C) as shown in Fig. 2a . Even at a rate of 13,790 mA g −1 (~8 C), cell capacity exceeds 450 mAh g −1 , demonstrating exceptional rate performance. In addition, marked improvement in capacity retention after repeated cycling is observed ( Fig. 2b ). 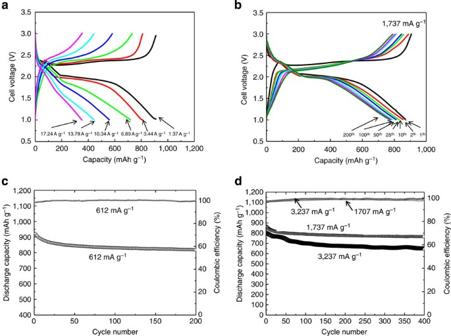Figure 2: Electrochemical behaviours of Li–S cells using the proposed hybrid anode. (a) Charge–discharge curves of hybrid Li–S cells at different rates. (b) Cycling ability of the hybrid Li–S cell at a rate of 1,737 mA g−1. (c,d) Long-term cycling behaviour and corresponding Coulombic efficiencies of hybrid Li–S cells at different rates. Figure 2c,d compares the long-term cycling behaviour and Coulombic efficiency of Li–S cells containing hybrid anode at different current density. Significantly improved cycling stability has been observed at all rates. For example, at 612 mA g −1 , the discharge capacity becomes stable after 50 cycles, maintaining at ~850 mAh g −1 for >200 cycles with a small initial capacity loss. The Columbic efficiency is always >99.5% over the entire cycling test ( Fig. 2c ), reflecting that the shuttle mechanism is significantly mitigated in this fundamentally different design of Li–S cells. Similar performance enhancements were observed at increased rates and over longer cycling times ( Fig. 2b,d ), strongly suggesting that this innovative anode concept plays a key role in extending the cycling life of this system. At 1,737 mA g −1 , the hybrid Li–S cell retains a capacity of >800 mAh g −1 after 400 cycles, corresponding to only 11% fade and a Coulombic efficiency of >99%. The electrochemical performances of Li–S batteries without hybrid anode design but using the same sulphur cathode are also included in Supplementary Information for comparison ( Supplementary Fig. S1 ). Figure 2: Electrochemical behaviours of Li–S cells using the proposed hybrid anode. ( a ) Charge–discharge curves of hybrid Li–S cells at different rates. ( b ) Cycling ability of the hybrid Li–S cell at a rate of 1,737 mA g −1 . ( c , d ) Long-term cycling behaviour and corresponding Coulombic efficiencies of hybrid Li–S cells at different rates. Full size image Materials characterization The cycled anode was further investigated after extensive cycling (Fig. 3). Energy dispersive spectroscopy, X-ray diffraction and X-ray photoelectron spectroscopy uncover that the chemical composition on Li metal surface in traditional Li–S cells is complex and comprises sulphide, sulphate, fluoride and carbonate compounds (Supplementary Fig. S2). Unlike the traditional SEI film formed on the anode surface, the chemical composition of surface film on the anode for Li–S batteries is more sophisticated, as ether-based solvents have been used and polysulphides get involved in the SEI growth [51] . Continued reactions between Li and dissolved polysulphide create an unstable reaction zone that comprises complicated sulphur-containing chemicals, lowering the Coulombic efficiency ( Supplementary Fig. S1 ). Similar SEI composition is expected on graphite surface, as in the same solution their surface chemistry is quite similar to each other [52] . The surface of Li metal harvested from the hybrid electrode remains relatively clean and free of polysulphide deposits. Careful compositional and structural analysis on the cycled hybrid anode suggests that although some polysulphides are deposited on the graphite surface ( Fig. 3c and Supplementary Fig. S3 ), the undesired parasitic reactions and accompanying sulphur contamination is greatly decreased on the Li metal ( Fig. 3d–f ). In contrast, the Li anode dissembled from traditional cycled Li–S batteries witnessed a large amount of S-containing species not only on Li metal surface but deeply penetration into bulk Li ( Fig. 3g–i ). 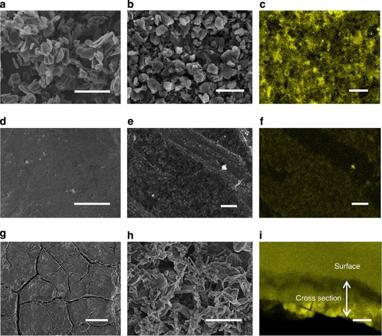Figure 3: Microstructure characterization of the hybrid anode. Scanning electrom microscopy (SEM) images of (a) native graphite and (b) graphite anode harvested from the hybrid anodes in Li–S cells after 1,000 cycles, respectively. (c) Sulphur elemental mapping on graphite anode obtained from the hybrid anodes after 1,000 cycles. (d,e) SEM images of the surface view of Li metal anode from the hybrid anodes after 1,000 cycles at different magnifications. (f) Sulphur elemental mapping of Li metal surface from the hybrid anodes after 1,000 cycles. The current density used for the 1,000 cycles was 3,237 mA g−1. (g,h) SEM images of the surface view of Li metal anode from traditional Li–S cells after 1,000 cycles at different magnifications. (i) S-elemental mapping of the Li metal anode from traditional Li–S cells. The current density used for the 1,000 cycles was 2,042 mA g−1. Scale bar, 50 μm (a–c,g,i), 40 μm (d), 10 μm (e,f) and 3 μm (h). Figure 3: Microstructure characterization of the hybrid anode. Scanning electrom microscopy (SEM) images of ( a ) native graphite and ( b ) graphite anode harvested from the hybrid anodes in Li–S cells after 1,000 cycles, respectively. ( c ) Sulphur elemental mapping on graphite anode obtained from the hybrid anodes after 1,000 cycles. ( d , e ) SEM images of the surface view of Li metal anode from the hybrid anodes after 1,000 cycles at different magnifications. ( f ) Sulphur elemental mapping of Li metal surface from the hybrid anodes after 1,000 cycles. The current density used for the 1,000 cycles was 3,237 mA g −1 . ( g , h ) SEM images of the surface view of Li metal anode from traditional Li–S cells after 1,000 cycles at different magnifications. ( i ) S-elemental mapping of the Li metal anode from traditional Li–S cells. The current density used for the 1,000 cycles was 2,042 mA g −1 . Scale bar, 50 μm ( a – c , g , i ), 40 μm ( d ), 10 μm ( e , f ) and 3 μm ( h ). Full size image Graphite loading At first glance, hybrid anode in its current form ( Fig. 1 ) may affect the energy density of the whole cell, as it incorporates additional accessory weights. However, it was found that the ratio between sulphur and graphite also directly influences the cycling stability ( Supplementary Fig. S4 ). That is, the higher the S/LiC 6 ratio (thinner graphite), the more stable the cycling. In other words, to fully utilize the hybrid concept, the weight of graphite needs to be minimized while the sulphur loading has to be maximized. The weight burden from graphite is therefore largely reduced. Neither gravimetric nor volumetric energy densities of the whole Li–S battery adopting the hybrid anode will be influenced significantly. The exact mechanisms controlling the hybrid electrode are still under investigation. One possible explanation is that the lithiated graphite may function as a physical barrier that decreases the contact area of soluble species in the electrolyte with Li metal. Physical absorption of polysulphide species on graphite may reduce transport of soluble intermediates to the Li anode. Control cells were assembled in which the Li foil and graphite electrodes were not electrically connected, although geometrically identical to the hybrid anode connected in series. When compared with traditional Li–S cells ( Supplementary Fig. S1 ), there is a slight improvement in the cycling stability ( Supplementary Fig. S5 ), indicating that the graphite does form a physical barrier that retards polysulphide transport, but the effect is minimal. Once connected with Li metal, the lithiated graphite goes beyond that of a simple diffusion barrier as discussed earlier. This hybrid anode design also differentiates from prelithiated graphite anode. Data collected on a simple LiC 6 /S full cell, using the same sulphur cathode but with a prelithiated graphite anode (without any Li foil connected), show poor electrochemical performance (Supplementary Fig. S6), further indicating that the synergistic effect of the connected LiC 6 and Li metal anode is essential for performance enhancement [49] . When graphite is replaced by hard carbon ( Supplementary Fig. S7 ), the performance of the Li–S cell is clearly inferior to that obtained from the cell using original a LiC 6 /Li hybrid design. The lithiation/delithiation of hard carbon occurs over a much wide voltage range. This result suggests that it is likely to be that the hybrid anode may require an intercalation compound with an operating voltage close to that of Li metal to timely respond to the Li + extraction from the hybrid anode during charge. In addition, side reactions caused by the interactions between polysulphides and highly reductive Li occur throughout the whole electrochemical processes, as soluble polysulphides are generated in the beginning of the discharge and at the end of charge, which inevitably get involved in the SEI formation on the anode. The largely increased surface area of hard carbon nanowires (surface area: 75.8 m 2 g −1 ) compared with that of graphite (surface area: 6.4 m 2 g −1 ) provides more reactive sites for the parasitic reactions to initiate, weakening the hybrid anode effect, as can be reflected by the decreased Coulombic efficiency ( Supplementary Fig. S7 ). Of note, the reduced performance of the hard carbon-containing anode is still a large improvement over a traditional Li–S cell construction ( Supplementary Fig. S1 ). From the above discussion, the function of the hybrid design is beyond that of a simple physical barrier. It involves an artificial and stable surface with a lithiation/delithiation voltage close to that of the Li metal and the needs to maintain the pseudo-equal potential through the shorted circuit. Findings to date suggest the lithiated graphite in the hybrid system functions similar to an ‘artificial SEI layer’. Lithiated graphite negatives operate at a voltage only ~150 mV higher than that of Li metal. Theoretically, during discharge of Li–S cells, Li + ions should first be extracted from Li metal instead of lithiated graphite (LiC 6 ). When shorted to Li metal, the lithiated graphite and the Li anode should be at equal potential. The charge/discharge rates used in this work are substantially higher than those used in conventional LIBs. Li + ions will be released from both LiC 6 and Li metal simultaneously, because the surface concentration of Li + ions around either surface is very low (close to zero) at such high current densities. Under this condition, the slight voltage difference is negligible and Li + ion contributions to the electrolyte may be largely from lithiated graphite—considering its physical location in the cell configuration. As graphite is always connected to Li metal, once Li + is removed from graphite the Li + cations will be automatically ‘refilled’ from the Li metal sink to eliminate the potential difference. In other words, lithiated graphite may function as a dynamic ‘pump’ that concurrently ejects Li + ions on demand to the working electrode and drains Li + ions from the Li metal reservoir to reload the graphite layers concurrently. Now that the function of lithiated graphite during discharge has been discussed, what happens during charge needs to be considered. One major concern during charge is whether the Li + ions will deposit on Li metal or lithiated graphite. At high charge rates, overlithiation, or Li plating, on the graphite has been reported [53] . In the hybrid anode design, it is expected that Li+ ions plate on both graphite and Li surface during charge. However, the relative amount of deposited Li on graphite and Li probably depends on the current density and the cell chemistry. In the presence of dissolved polysulphides, the composition of SEI on graphite is more complicated than in traditional cells, as it contains insulating sulphur species ( Supplementary Fig. S3 ). The surface conductivity of lithiated graphite is lower than that of Li metal due to the existence of more insulating S-containing species on graphite film in the hybrid configuration. This is supported by the higher overpotential of Li deposition on lithiated graphite than on Li metal ( Supplementary Fig. S8 ). Therefore, the overplating of Li on graphite surface is largely reduced. In addition, multiple studies have shown that sulphur-containing electrolytes help eliminate dendritic spikes on the graphite surface by chemically etching the protuberant Li [46] , [53] , [54] . Therefore, in the hybrid design, the graphite functions as a ‘self-regulating’ shuttle, which significantly reduces unwanted side reactions on the Li metal surface during both discharge and charge. It has to be pointed out that the reduced side reactions on Li side mainly refers to the interactions between polysulphides and highly reductive Li, which continuously ‘consume’ active sulphur by forming a series of sulphur-containing byproducts ( Supplementary Figs S2 and S3 ). The continuous consumption of active sulphur and formation of S-containing byproducts happen only when the microstructure of Li metal continues to grow. If there is no microstructure evolution such as porous structure formed from dendritic Li during cycling, the accumulation of those S-based byproducts will be largely limited to the surface instead of deeply penetrating into the interior of the Li metal. Therefore, the structure evolution of Li metal anode will help to understand how the hybrid anode works to prevent side reactions. With this in mind, we studied the structure evolution of Li metal anode using symmetric cells. Supplementary Fig. S9 shows that protected Li anode (hybrid Li anode) had much more dense structure (without dendrite) on the surface after cycling than that of unprotected one (with dendrite) in the symmetric cells, and that electrolyte decomposition still occurs on Li metal but is largely alleviated in the presence of the graphite film. In this hybrid anode design, the shuttle reaction still exists on graphite anode; thus, LiNO 3 additive is still used in the electrolyte. However, the undesired reactions will not continuously grow, as the volume expansion of graphite is limited. On the basis of these discussions, there are at least two basic requirements that have to be satisfied for the hybrid anode design. First, the electrochemically formed artificial SEI takes advantage of intercalation chemistry. Intercalation compound such as graphite undergoes minimum volume expansion (up to 10%) during lithiation [55] . On repeated cycling, there is no structural damage on the graphite electrode that may expose new surfaces as parasite reaction sites. Second, minimum difference in operating voltages between the artificial SEI (lithiated graphite in this case) and Li metal ensures the timely refill of Li + ions into graphite lattice during the discharge process of Li–S batteries (extraction of Li + from anode). In summary, a radically different hybrid design has been introduced for Li–S cells to mitigate the loss of active material and harmful parasitic reactions on the anode by using an integrated structure composed of electrically connected graphite and Li metal. Although further studies are required, preliminary findings, combined with available literature results, support the idea that lithiated graphite functions as an electrochemical artificial SEI that decouples the Li + extraction/reinsertion from side reactions caused by soluble polysulphides. The anode reaction front is shifted from the Li metal to the graphite surface and the interaction with dissolved polysulphide species is primarily confined to graphite. The reduced irreversible sulphur loss on the Li metal anode, as well as the physical barrier benefit provided by the lithiated graphite, collectively leads to the exceptional electrochemical performances observed in Li–S batteries. This simple hybrid concept provides important clues in the future development of Li–S batteries and may be broadly adapted in many energy-storage technologies utilizing metal anodes. Cathode A mesoporous carbon-sulphur (MCS) nanocomposite was used for both hybrid Li–S cell and traditional Li–S cell cathodes. The MCS composite contains an mesoporous carbon with a large pore volume (22 nm, 4.8 cm 3 g −1 ) and controllable sulphur loading (50 wt%) [20] . The cathode was prepared by mixing 80 wt% MCS nanocomposite powder, 10 wt% Super-P Li conductive carbon black (TIMCAL, Graphite & Carbon Ltd) and 10 wt% polyvinylidene fluoride (Kynar HSV900, Arkema Inc.) binder in N -methylpyrrolidone onto aluminum foils and then dried at 55 °C for 12 h. Hybrid anode TIMREX SLP30 graphite powder (TIMCAL, Graphite & Carbon Ltd) was mixed with Super-P (Timcal) and polyvinylidene fluoride in a ratio of 8:1:1 in N -methylpyrrolidone. The slurry was then coated onto porous stainless steel mesh and then connected with the Li metal foil. A piece of Celgard 2400 was placed in between the graphite film and Li metal to form the hybrid anode for Li–S cells. It is critical that bonding fine metal filaments with carbon forms an interlocking composite network. The porous carbon–metallic grid composite electrode without carbon delamination or pinholes provides improved continuity of electrical conductivity and, hence, diminished Equivalent Series Resistance and advantageous modification of the macro-equivalent circuit. Cell assembly All of the coin cells (Type 2325 coin cell kits from CNRC, Canada) were assembled in an argon-filled glove box (MBraun, Inc.) with moisture and oxygen content of <1 p.p.m. Li metal disks were used as the anode. The electrolyte was 1 M bis(trifluoromethane) sulphonimide Li salt (99.95% trace metals basis, Sigma-Aldrich) dissolved in a mixture of 1,3-dioxolane (Sigma-Aldrich) and dimethoxymethane (Sigma-Aldrich; 1: 1 by volume). The dried and argon-protected LiNO 3 (Sigma-Aldrich) additive was then added into the electrolyte to reach a concentration of 0.1 M. Electrochemical tests Electrochemical tests were performed using 2,325 coin cells (NRC, Canada) in ambient environment. The galvanostatic discharge–charge test was conducted using a BT-2043 Arbin Battery Testing System. All the cells were cycled at different current rates in the voltage interval of 1.0–3.0 V. All capacity values were calculated on the basis of sulphur mass. After cycling, several of the coin cells were disassembled in the charged or discharged state for further analysis. Electrode characterization To analyse the electrode properties and cell operation mechanisms, several of the coin cells were disassembled in the fresh, discharged or charged state, respectively. Each electrode, including Li anode, carbon anode and MCS cathode, was thoroughly washed in the glove box by a mixture solvent of 1,3-dioxolane and dimethoxymethane (1:1 by volume) to remove any electrolyte salt residuals, and then transferred into vacuum chamber via a Sample Saver storage container (South Bay Technology, Inc.). Scanning electron microscopy experiments for the investigation of the electrode surface morphology and composition were performed on an FEI Quanta 3D FEG focused ion beam/scanning electron microscope equipped with an Oxford INCA PentFEXx3 system with 33 mm window EDAX detector. For quantitative comparison of S-elemental contents of Li anode surfaces from the half cell and full cell, S-elemental mapping with fixed frame collection counts (Res: 256 × 200 and Frame Reads: 500/500) was used to calculate atom% of S K versus atom% of C K. X-ray photoelectron spectroscopy measurements were performed with a Physical Electronics Quantera Scanning X-ray Microprobe. This system uses a focused monochromatic Al K α X-ray (1,486.7 eV) source for excitation and a spherical section analyser. The instrument has a 32-element multichannel detection system. A 100-W X-ray beam focused to 100 μm diameter was rastered over a 1.4 × 0.1 mm rectangle on the sample. The X-ray beam is incident normal to the sample and the photoelectron detector is at 45° off-normal. High-energy resolution (narrow scan) X-ray photoemission spectra were collected using a pass energy of 69.0 eV with a step size of 0.125 eV. For the Ag 3d5/2 line, these conditions produced a full width at half maximum of 0.91 eV. The sample experienced variable degrees of charge. All the spectra were charge referenced using C 1 s line at 285.0 eV for comparison purpose. Low-energy electrons at ~1 eV, 20 μA and low-energy Ar + ions were used to minimize this charge. How to cite this article: Huang, C. et al. Manipulating surface reactions in lithium–sulphur batteries using hybrid anode structures. Nat. Commun. 5:3015 doi: 10.1038/ncomms4015 (2014).